Ulk1-mediated Atg5-independent macroautophagy mediates elimination of mitochondria from embryonic reticulocytes Macroautophagy is a highly conserved intracellular process responsible for the degradation of subcellular constituents. Macroautophagy was recently suggested to be involved in the removal of mitochondria from reticulocytes during the final stage of erythrocyte differentiation. Although Atg5 and Atg7 are indispensable for macroautophagy, their role in mitochondrial clearance remains controversial. We recently discovered that mammalian cells use conventional Atg5/Atg7-dependent macroautophagy as well as an alternative Unc-51-like kinase 1 (Ulk1)-dependent Atg5/Atg7-independent macroautophagy process. We hypothesized that the latter may be involved in mitochondrial clearance from reticulocytes during erythrocyte differentiation. Here we report that fetal definitive reticulocytes from Ulk1-deficient and Ulk1/Atg5 double-deficient mice retain their mitochondria, whereas the mitochondria are engulfed and digested within autophagic structures in wild-type and Atg5-deficient mice. Mitochondrial retention by Ulk1-deficient reticulocytes is far less marked in primitive and adult definitive reticulocytes. These data indicate that Ulk1-dependent Atg5-independent macroautophagy is the dominant process of mitochondrial clearance from fetal definitive reticulocytes. Macroautophagy is an essential maintenance and protective catabolic process involving the digestion of cellular components and damaged organelles within the lysosomes [1] , [2] . Macroautophagy occurs constitutively at a low level, but is accelerated by cellular stressors, such as starvation, lack of growth factors and DNA damage. The molecular basis of macroautophagy was extensively studied using autophagy-defective mutant yeasts and mammals [2] , [3] . It is currently accepted that macroautophagy is driven by >30 autophagy-related proteins (Atgs) conserved from yeasts to mammals [4] . The process of macroautophagy is initiated by the multiprotein complex phosphatidylinositol 3-kinase (PI3K) type III containing Atg6 (also called Beclin1), which promotes membrane invagination [5] . The subsequent elongation and closure of the isolation membrane is mediated by two ubiquitin-like conjugation pathways: the Atg5-Atg12 pathway and the microtubule-associated protein 1 light chain 3 (LC3) pathway [4] . Both pathways depend on the E1-like enzyme Atg7. Thus, several core macroautophagy molecules are believed to be indispensable for macroautophagy, particularly PI3K, Atg5 and Atg7. We recently discovered that macroautophagy occurs in cells lacking Atg5 and Atg7 (ref. 6 ). We named this process ‘alternative macroautophagy’ to distinguish it from Atg5/Atg7-dependent conventional macroautophagy. The role is similar to conventional macroautophagy; whereby, cellular components and organelles are digested within autophagosomes. But the signalling pathway involves PI3K, and not Atg5, Atg7 or LC3. We also found that this pathway is largely dependent on Unc-51-like kinase 1 (Ulk1), a mammalian homologue of yeast Atg1. This kinase is involved in the initiation of conventional macroautophagy and several regulatory mechanisms have been proposed. During starvation, the mTOR complex 1 dissociates from Ulk1, leading to Ulk1 dephosphorylation and activation of the UlK1-Atg13-FIP200-Atg101 complex [7] . In another pathway, Ulk1 is stabilized and activated by the Hsp90-Cdc37 complex [8] . Furthermore, it has been reported that Ulk1 is phosphorylated and acetylated by AMP-activated protein kinase (AMPK) [9] and Tip60 (ref. 10 ), respectively. All of the above reports were related to the mechanisms by which Ulk1 initiates conventional macroautophagy. However, cells from Ulk1-knockout mice maintained low but significant macroautophagy activity [11] . This study suggests that Ulk1 is not essential for conventional Atg5/Atg7-dependent macroautophagy, but improves the efficiency [11] . This kinase was upregulated during alternative macroautophagy, and Ulk1 silencing markedly inhibited the alternative process [6] . Therefore, Ulk1 may have a dual role, as a facilitator of conventional macroautophagy and as an essential trigger for alternative macroautophagy. Macroautophagy was previously considered to be a nonselective process, but recent studies demonstrated that distinct macroautophagy signalling pathways regulate the digestion of specific organelles [12] , [13] . During erythrocyte maturation, the erythroblasts lose their nuclei to become reticulocytes, which are transformed into erythrocytes (EC) by the elimination of organelles, including the mitochondria. It is believed that macroautophagy is involved in this process because ultrastructural studies have detected autophagic structures engulfing mitochondria [14] , [15] . The involvement of Atg5 and Atg7 remains controversial due to conflicting reports [16] , [17] , [18] . In contrast, Ulk1 has been reported to have an important role [8] , [11] . Therefore, we hypothesized that mitochondrial clearance during erythrocyte maturation may be performed by Ulk1-dependent Atg5-independent alternative macroautophagy. This hypothesis was tested by studying mitochondrial clearance from fetal definitive reticulocytes from Ulk1-deficient, Atg5-deficient and Ulk1/Atg5 double-deficient mouse embryos. The contribution of alternative macroautophagy was determined on the basis of the difference between the Atg5-deficient embryos and Ulk1/Atg5 double-deficient embryos. We also determined the weak involvement of Ulk1 in mitochondrial clearance from primitive and adult definitive reticulocytes. Our findings indicate that Ulk1-dependent Atg5-independent macroautophagy is the dominant pathway for mitochondrial clearance from fetal definitive reticulocytes, whereas its role is less important in primitive and adult definitive reticulocytes. Generation of Ulk1-deficient and Atg5/Ulk1-deficient mice Ulk1-deficient mice were generated from embryonic stem cells by inserting a gene-trap in ulk1 ( Supplementary Fig. 1a ). The absence of Ulk1 protein in the hematopoietic cells of Ulk1 gt/gt mice was verified by western blotting ( Fig. 1a ). The Ulk1 gt/gt mice showed mild anaemia ( Supplementary Fig. 1b ) and splenomegaly ( Supplementary Fig. 1c ), consistent with the phenotype of Ulk1 −/− mice [11] . In addition, Ulk1/Atg5 double-deficient (DKO) mice were generated by crossbreeding Ulk1 gt/gt mice with Atg5 +/− mice ( Fig. 1a ). The terminal differentiation of EC proceeded normally in Ulk1 gt/gt , Atg5 −/− and DKO mice, as assessed by the expression of Ter119 and CD71 ( Supplementary Fig. 2 ). These markers were used to identify the different maturation stages of erythroid cells into EC. 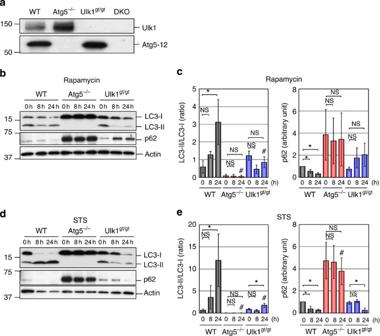Figure 1: Induction of conventional macroautophagy in Atg5-deficient erythroid cells by rapamycin and STS. (a) Expression of Ulk1 and Atg5–12 in the indicated erythroid cells. (b–e) Induction of conventional macroautophagy in WT and Ulk1gt/gt, but not in Atg5−/−, embryonic erythroid cells. Ter119+erythroid cells from WT, Atg5−/−, and Ulk1gt/gtembryonic mice (E18.5) were treated with 1 μM rapamycin (b,c) and 1 μM STS (d,e), and then harvested at the indicated times. (b,d) Representative protein expression of LC3 and p62 measured by western blot. Actin was a loading control. Uncropped images are shown inSupplementary Fig. 10. (c,e) Semi-quantitative analysis of LC3-II/LC3-I and p62 protein expression (n=3, mean±s.d.). Asterisks indicate a significant difference atP<0.05 (analysis of variance (ANOVA)).#P<0.05 versus value of WT 24 h (ANOVA). ‘NS’ indicates not significant (ANOVA). Figure 1: Induction of conventional macroautophagy in Atg5-deficient erythroid cells by rapamycin and STS. ( a ) Expression of Ulk1 and Atg5–12 in the indicated erythroid cells. ( b – e ) Induction of conventional macroautophagy in WT and Ulk1 gt/gt , but not in Atg5 −/− , embryonic erythroid cells. Ter119 + erythroid cells from WT, Atg5 −/− , and Ulk1 gt/gt embryonic mice (E18.5) were treated with 1 μM rapamycin ( b , c ) and 1 μM STS ( d , e ), and then harvested at the indicated times. ( b , d ) Representative protein expression of LC3 and p62 measured by western blot. Actin was a loading control. Uncropped images are shown in Supplementary Fig. 10 . ( c , e ) Semi-quantitative analysis of LC3-II/LC3-I and p62 protein expression ( n =3, mean±s.d.). Asterisks indicate a significant difference at P <0.05 (analysis of variance (ANOVA)). # P <0.05 versus value of WT 24 h (ANOVA). ‘NS’ indicates not significant (ANOVA). Full size image Induction of Ulk1-dependent mitophagy by staurosporine The wild-type (WT), Ulk1 gt/gt and Atg5 −/− mice were first tested for the presence of functional conventional and/or alternative macroautophagy in cells of the erythroid lineage. The cells were harvested from the liver of embryonic mice on day 18.5 (E18.5) using microbeads conjugated with anti-Ter119 antibodies. The cells were treated with rapamycin to selectively induce conventional (not alternative) macroautophagy [6] , and examined for the lipid conjugation of microtubule-associated protein LC3 that occurs during conventional (but not alternative) macroautophagy [6] . LC3-II (a lipid conjugate) was observed in WT cells, but not in Atg5 −/− cells, after rapamycin treatment ( Fig. 1b,c ). Lesser LC3-II formation was detected in Ulk1 gt/gt cells than in WT. We also examined the expression of p62, a specific substrate of conventional macroautophagy. Consistent with LC3-II formation, the highest expression of p62 was found in Atg5 −/− cells, followed by Ulk1 gt/gt and WT cells ( Fig. 1b,c ). Similar results were obtained when these cells were treated with staurosporine (STS), a pan-kinase inhibitor ( Fig. 1d,e ). These results show that the lack of Ulk1 expression partially inhibited conventional macroautophagy in erythroid cells. Conventional and alternative macroautophagy were visualized by confocal microscopy using the non-selective autophagy inducer STS and antibodies against lysosomal-associated membrane protein 2 (Lamp2). Lysosomes are small vesicles distributed throughout the cytosol, so that Lamp2 fluorescence is seen as tiny dots. After the induction of macroautophagy, lysosomes fuse with autophagic vacuoles and the area of Lamp2 fluorescence become much larger. Thus, large Lamp2 fluorescence dots are identical to autolysosomes, as described previously [6] . Small diffuse fluorescent dots were observed in untreated WT erythroid cells, whereas STS-treated WT erythroid cells contained large fluorescent dots ( Fig. 2a ) suggestive of macroautophagy induction. Large fluorescent dots similar in size and number were observed in STS-treated Atg5 −/− erythroid cells. Because conventional macroautophagy was not induced in these cells, the large Lamp2 dots suggest that STS induced alternative macroautophagy. In contrast, fewer large Lamp2 dots were detected in STS-treated Ulk1 gt/gt and STS-treated Ulk1 gt/gt Atg5 −/− DKO erythroid cells, suggesting that Ulk1 is involved in both conventional and alternative macroautophagy. 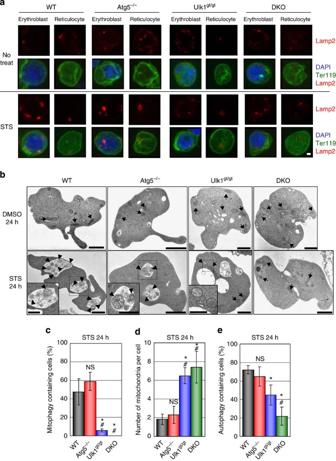Figure 2: Induction of alternative macroautophagy in Atg5-deficient erythroid cells by STS. (a) Induction of alternative macroautophagy in WT and Atg5−/−, but not Ulk1gt/gtand DKO, erythroid cells. Erythroblasts and reticulocytes from the liver of embryonic mice (E18.5) were incubated with or without STS (1 μM) for 24 h, followed by staining with anti-Lamp2 (red), anti-Ter119 (green) and DAPI (blue). DAPI-positive erythroblasts and DAPI-negative reticulocytes are shown. Lamp2 image and merged image (DAPI, Ter119 and Lamp2) are shown. Scale bar, 1 μm. Large dots for Lamp2 are observed in STS-treated WT and Atg5−/−cells, but not STS-treated Ulk1gt/gtor DKO cells. (b) Representative electron micrographs of EC incubated with or without STS. Erythroid cells were harvested from the liver of embryonic mice (E18.5), incubated with or without STS (1 μM) for 24 h, and analysed by electron microscopy (EM). Scale bar, 1 μm. Insets of WT and Atg5−/−cells show mitophagy (Scale bar, 0.5 μm). Inset of a Ulk1gt/gtcell showing mitochondria that have not been engulfed (Scale bar, 0.5 μm). Arrows point to non-engulfed mitochondria and the arrowheads indicate engulfed mitochondria. (c–e) Quantitative analysis of mitophagy after STS treatment, calculated from EM photos. Population of reticulocytes with mitophagy (c), number of mitochondria per reticulocytes (d) and population of reticulocytes showing macroautophagy (e) were calculated (n>35 cells per mouse). The data are shown as mean±s.d. (n=3). *P<0.05 versus value of WT (analysis of variance (ANOVA));#P<0.05 versus value of Atg5−/−(ANOVA); ‘NS’ indicates not significant versus value of WT (ANOVA). Figure 2: Induction of alternative macroautophagy in Atg5-deficient erythroid cells by STS. ( a ) Induction of alternative macroautophagy in WT and Atg5 −/− , but not Ulk1 gt/gt and DKO, erythroid cells. Erythroblasts and reticulocytes from the liver of embryonic mice (E18.5) were incubated with or without STS (1 μM) for 24 h, followed by staining with anti-Lamp2 (red), anti-Ter119 (green) and DAPI (blue). DAPI-positive erythroblasts and DAPI-negative reticulocytes are shown. Lamp2 image and merged image (DAPI, Ter119 and Lamp2) are shown. Scale bar, 1 μm. Large dots for Lamp2 are observed in STS-treated WT and Atg5 −/− cells, but not STS-treated Ulk1 gt/gt or DKO cells. ( b ) Representative electron micrographs of EC incubated with or without STS. Erythroid cells were harvested from the liver of embryonic mice (E18.5), incubated with or without STS (1 μM) for 24 h, and analysed by electron microscopy (EM). Scale bar, 1 μm. Insets of WT and Atg5 −/− cells show mitophagy (Scale bar, 0.5 μm). Inset of a Ulk1 gt/gt cell showing mitochondria that have not been engulfed (Scale bar, 0.5 μm). Arrows point to non-engulfed mitochondria and the arrowheads indicate engulfed mitochondria. ( c – e ) Quantitative analysis of mitophagy after STS treatment, calculated from EM photos. Population of reticulocytes with mitophagy ( c ), number of mitochondria per reticulocytes ( d ) and population of reticulocytes showing macroautophagy ( e ) were calculated ( n >35 cells per mouse). The data are shown as mean±s.d. ( n =3). * P <0.05 versus value of WT (analysis of variance (ANOVA)); # P <0.05 versus value of Atg5 −/− (ANOVA); ‘NS’ indicates not significant versus value of WT (ANOVA). Full size image The two types of macroautophagy were distinguished using anti-LC3 antibodies because this protein only associates with autolysosomes during conventional macroautophagy, and therefore is a good marker to distinguish these two types of autophagic machineries. In this assay, the addition of a lysosomal protease inhibitor (E64d) was required to prevent LC3 degradation in autolysosomes. Selective induction of conventional macroautophagy with rapamycin generated only LC3-positive Lamp2 dots in WT cells ( Supplementary Fig. 3 ). In contrast, STS-treated Atg5 −/− cells, where alternative macroautophagy was selectively generated, contained only LC3-negative Lamp2 dots ( Supplementary Fig. 3 ). Expectedly, STS-treated WT and Ulk1 gt/gt cells possessed both types of Lamp2 dots. In addition, the size and number of Lamp2 dots was significantly lower in Ulk1 gt/gt cells ( Supplementary Fig. 3 ). These findings suggest that STS induces conventional and alternative macroautophagy, both of which are largely dependent on Ulk1. The process of STS-mediated macroautophagy in erythroid cells was further examined by electron microscopy. In WT cells, this exposure caused the formation of several large autophagic vacuoles. The vacuoles engulfed cytoplasmic constituents and mitochondria. Erythroid cells may be unusually susceptible to mitochondrial digestion by macroautophagy (‘mitophagy’) because this phenomenon was rarely observed in STS-treated embryonic fibroblasts. Similar autophagic vacuoles were observed in Atg5 −/− erythroid cells, but not in DKO erythroid cells ( Fig. 2b ). Quantitative analysis revealed that mitophagy occurred in about 50% of WT cells and 60% of Atg5 −/− cells ( Fig. 2c ), and the number of mitochondria among these cells was low ( Fig. 2d ). Autophagic vacuoles were also observed in STS-treated Ulk1 gt/gt cells ( Fig. 2b,e ), but most of them were not used for mitophagy. Thus, the cell population exhibiting mitophagy was small ( Fig. 2c ), and the number of mitochondria in STS-treated Ulk1 gt/gt cells was higher than in STS-treated WT or STS-treated Atg5 −/− cells ( Fig. 2d ). DKO cells contained only a few autophagic vacuoles ( Fig. 2b,e ), and the mitochondrial numbers were high ( Fig. 2d ). Although STS is a well-known apoptosis inducer, the apoptotic cell population was low (<25%) under these conditions ( Supplementary Fig. 4a ). Furthermore, the apoptosis inhibitor Qvd-fmk did not significantly alter the extent of mitochondrial clearance ( Supplementary Fig. 4b ), indicating that apoptosis was not involved in macroautophagy and mitochondrial clearance. Altogether, these findings indicate that STS induces both conventional and Ulk1-dependent alternative macroautophagy in erythroid cells, and that mitochondria are mainly removed by the latter. Mitochondrial removal by alternative macroautophagy in vivo Experiments were designed to determine the role of Ulk1-dependent alternative macroautophagy in mitochondrial clearance during erythrocyte differentiation. Hematopoietic ontogeny includes three waves of erythroid lineage: primitive, fetal definitive and adult definitive. The existence of this process in fetal definitive erythroid cells was assessed. Three-colour flow cytometric analysis was conducted using a marker of erythroid precursors (CD71), a marker of late stage erythroid lineage (Ter119) and mitochondria-specific Mitotracker Deep Red staining, indicating that nearly all CD71 + Ter119 − cells ( Fig. 3a left upper panel; R1 fraction) and CD71 + Ter119 + cells ( Fig. 3a left upper panel; R2 fraction) showed strong Mitotracker staining ( Fig. 3a right upper and left lower panels) in erythroid cells harvested from the liver of WT embryos on E14.5. In contrast, about 60% of the CD71 − Ter119 + cells (mature EC) showed weak Mitotracker staining ( Fig. 3a left upper panel; R3 fraction, Fig. 3a right lower panel) due to mitochondrial clearance during differentiation. The cell population containing low numbers of mitochondria (mitochondria low cells) among mature Atg5 −/− EC ( Fig. 3b,c ; E14.5 Atg5 −/− ) was equivalent to that of mature WT EC ( Fig. 3b,c ; E14.5 WT). This population was smaller in Ulk1 gt/gt and DKO EC ( Fig. 3b,c ; E14.5 Ulk1 gt/gt and DKO). These data show that erythrocyte differentiation requires Ulk1, but not Atg5, for mitochondrial clearance on E14.5. 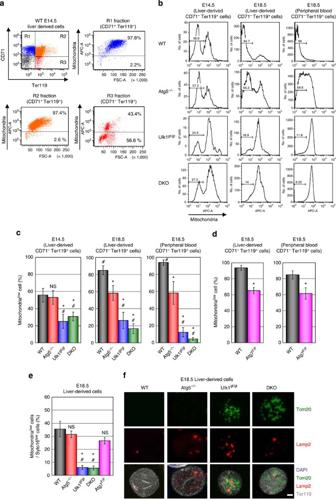Figure 3: Impaired clearance of mitochondria in Ulk1gt/gtand DKO EC. (a) Three-colour flow cytometry of erythroid cells from WT embryonic liver (E14.5) stained with anti-Ter119, anti-CD71 and Mitotracker Deep Red. (Left upper panel) Ter119 versus CD71 fluorescence. (Other panels) FSC versus Mitotracker fluorescence of the R1 (right upper panel), R2 (left lower panel) and R3 (right lower panel) fractions. (b,c) Percentage of cells with a low number of mitochondria (mitochondrialowcells) among CD71−Ter119+EC. Erythroid cells from the liver (E14.5 and E18.5) and peripheral blood (E18.5) of indicated mice were stained with anti-Ter119, anti-CD71 and Mitotracker Deep Red. (b) Representative histograms of mitochondrial content in CD71−Ter119+cells. Numbers indicate the population of mitochondrialowcells. (c) The percentage of CD71−Ter119+cells without mitochondria was determined by gating the mitochondrialowfraction, as shown in (b) (mean±s.d.,n=6). *P<0.05 versus value of WT (analysis of variance (ANOVA));#P<0.05 versus value of Atg5−/−(ANOVA); ‘NS’ indicates not significant versus value of WT (ANOVA). (d) Percent mitochondrialowcells in the CD71−Ter119+EC of Atg7F/FCre embryo. Erythroid cells from the liver and peripheral blood of WT and Atg7F/FCre embryo (E18.5) were stained with anti-Ter119, anti-CD71, and Mitotracker Deep Red (mean±s.d.,n=3). *P<0.05 versus value of WT (Student'st-test). (e) Percentage of mitochondrialowcells in Syto16lowcells. Liver erythroid cells (E18.5) were stained with Syto16 (DNA) and Mitotracker Deep Red. Representative dot plots of the mitochondrial content of Syto16lowcells are demonstrated inSupplementary Fig. 5, the percentage of Syto16lowcells without mitochondria was determined by gating the mitochondrialowfraction (mean±s.d.,n=6). *P<0.05 versus value of WT (ANOVA);#P<0.05 versus value of Atg5−/−(ANOVA); ‘NS’ indicates not significant versus value of WT (ANOVA). (f) Immunofluorescent analysis of mitochondrial and lysosomal proteins. Liver Ter119+cells (E18.5) of the indicated mice were stained with anti-Tom20 (mitochondrial marker) and anti-Lamp2 (lysosomal marker) antibodies, and observed by fluorescent microscopy. Scale bar, 2 μm. Green, red, white, and blue indicate Tom20, Lamp2, Ter119 and DAPI (DNA), respectively. Mitochondrial and lysosomal markers have separate distributions in Ulk1gt/gtcells and DKO cells. Figure 3: Impaired clearance of mitochondria in Ulk1 gt/gt and DKO EC. ( a ) Three-colour flow cytometry of erythroid cells from WT embryonic liver (E14.5) stained with anti-Ter119, anti-CD71 and Mitotracker Deep Red. (Left upper panel) Ter119 versus CD71 fluorescence. (Other panels) FSC versus Mitotracker fluorescence of the R1 (right upper panel), R2 (left lower panel) and R3 (right lower panel) fractions. ( b , c ) Percentage of cells with a low number of mitochondria (mitochondria low cells) among CD71 − Ter119 + EC. Erythroid cells from the liver (E14.5 and E18.5) and peripheral blood (E18.5) of indicated mice were stained with anti-Ter119, anti-CD71 and Mitotracker Deep Red. ( b ) Representative histograms of mitochondrial content in CD71 − Ter119 + cells. Numbers indicate the population of mitochondria low cells. ( c ) The percentage of CD71 − Ter119 + cells without mitochondria was determined by gating the mitochondria low fraction, as shown in ( b ) (mean±s.d., n =6). * P <0.05 versus value of WT (analysis of variance (ANOVA)); # P <0.05 versus value of Atg5 −/− (ANOVA); ‘NS’ indicates not significant versus value of WT (ANOVA). ( d ) Percent mitochondria low cells in the CD71 − Ter119 + EC of Atg7 F/F Cre embryo. Erythroid cells from the liver and peripheral blood of WT and Atg7 F/F Cre embryo (E18.5) were stained with anti-Ter119, anti-CD71, and Mitotracker Deep Red (mean±s.d., n =3). * P <0.05 versus value of WT (Student's t -test). ( e ) Percentage of mitochondria low cells in Syto16 low cells. Liver erythroid cells (E18.5) were stained with Syto16 (DNA) and Mitotracker Deep Red. Representative dot plots of the mitochondrial content of Syto16 low cells are demonstrated in Supplementary Fig. 5 , the percentage of Syto16 low cells without mitochondria was determined by gating the mitochondria low fraction (mean±s.d., n =6). * P <0.05 versus value of WT (ANOVA); # P <0.05 versus value of Atg5 −/− (ANOVA); ‘NS’ indicates not significant versus value of WT (ANOVA). ( f ) Immunofluorescent analysis of mitochondrial and lysosomal proteins. Liver Ter119 + cells (E18.5) of the indicated mice were stained with anti-Tom20 (mitochondrial marker) and anti-Lamp2 (lysosomal marker) antibodies, and observed by fluorescent microscopy. Scale bar, 2 μm. Green, red, white, and blue indicate Tom20, Lamp2, Ter119 and DAPI (DNA), respectively. Mitochondrial and lysosomal markers have separate distributions in Ulk1 gt/gt cells and DKO cells. Full size image In mature EC harvested from the liver and blood on E18.5, most WT cells no longer contained mitochondria ( Fig. 3b,c ; E18.5 WT), whereas <25% of Ulk1 gt/gt and DKO EC had lost their mitochondria ( Fig. 3b,c ; E18.5 Ulk1 gt/gt and DKO), indicating a failure to clear mitochondria in the absence of Ulk1. The mitochondria low population among mature Atg5 −/− EC was smaller than that among mature WT EC, but considerably larger than that among Ulk1 gt/gt and DKO EC ( Fig. 3b,c ; E18.5 Atg5 −/− ). Similar results were obtained with hematopoietic-specific Atg7 conditional knockout (Atg7 F/F ;vav1-cre (Atg7 F/F Cre)) mice ( Fig. 3d ). These data indicate that Ulk1 plays a predominant role, compared with that of Atg5 and Atg7, in mitochondrial clearance from reticulocytes on E18.5. During erythrocyte differentiation, mitochondria elimination is initiated after enucleation. Therefore, the efficiency of mitochondrial clearance was determined by staining cells with the DNA-specific stain Syto16 and Mitotracker Deep Red. Syto16 low cells identified enucleated cells, and the efficiency was calculated from the ratio of mitochondria low Syto16 low cells to the total amount of Syto16 low cells ( Supplementary Fig. 5 ). The population of mitochondria low Syto16 low EC was smaller in Ulk1 gt/gt and DKO embryos than in WT, Atg5 −/− and Atg7 F/F Cre embryos ( Fig. 3e ). These data are consistent with the results obtained by Ter119/CD71/Mitotracker staining ( Fig. 3c,d ). Furthermore, when late erythroid lineage Ter119-positive cells were immunostained with mitochondria-specific anti-Tom20 antibodies, positive signals were detected in most Ulk1 gt/gt and DKO EC, but only in a few WT and Atg5 −/− EC ( Fig. 3f ). Mitochondrial signals rarely merged with Lamp2 fluorescence in Ulk1 gt/gt and DKO EC, suggesting that mitophagy did not occur. Altogether, these data indicate that Ulk1 is considerably more important than Atg5 for mitochondrial clearance from reticulocytes during the embryonic period. The involvement of macroautophagy during the mitochondrial clearance from reticulocytes was further investigated on the basis of ultrastructural changes visualized by EM. On E14.5, the mitochondria was engulfed and digested by autophagic vacuoles in WT reticulocytes ( Fig. 4a ) and Atg5 −/− reticulocytes ( Fig. 4b ). The cell population exhibiting mitophagy was similar in these two types of reticulocytes ( Fig. 4g ), whereas mitophagy was largely suppressed in Ulk1 gt/gt reticulocytes ( Fig. 4c,g ). These findings are consistent with the data obtained by flow cytometry ( Fig. 3c,e ). In DKO reticulocytes, mitophagy was also markedly suppressed, compared with WT reticulocytes ( Fig. 4e,g ). Accordingly, the number of mitochondria remaining in Ulk1 gt/gt and DKO reticulocytes was larger than in WT and Atg5 −/− reticulocytes ( Fig. 4h ). Numerous mitochondria were in contact with the membranous structure in Ulk1 gt/gt and DKO reticulocytes. This may indicate that mitochondria were recognized by the isolation membrane, but not enclosed due to the lack of Ulk1. Some of the Ulk1 gt/gt and DKO reticulocytes formed plasma membrane blebs and shed cell fragments containing mitochondria ( Fig. 4d,f ), which may represent a process that removes undigested mitochondria. All these morphological findings support a predominant role for Ulk1-dependent Atg5-independent macroautophagy in the mitochondrial clearance from reticulocytes. 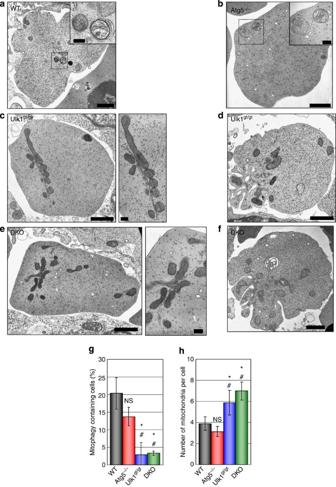Figure 4: Clearance of mitochondria by macroautophagy from reticulocytes of WT and Atg5−/−mice, but not Ulk1gt/gtor DKO mice. (a–f) Representative EM of WT (a), ATG5−/−(b), Ulk1gt/gt(c,d) and DKO (e,f) reticulocytes from embryonic liver (E14.5). (a,b) Mitophagy was detected in WT and ATG5−/−cells (scale bar, 1 μm). Insets indicate mitophagy (scale bar, 0.2 μm). (c,e) In Ulk1gt/gtand DKO cells, numerous mitochondria were in contact with membrane structures (scale bar, 1 μm). Enlarged images are shown on the right side (scale bar, 0.2 μm). (d,f) Some Ulk1gt/gtand DKO cells showed plasma membrane blebs containing mitochondria (scale bar, 1 μm). (g,h) Quantitative analysis of mitophagy calculated from EM photos in the embryonic liver at E18.5. Population of reticulocytes with mitophagy (g), and number of mitochondria per reticulocytes (h) were calculated (n>35 cells per mouse). The data are shown as mean±s.d. (n=3). *P<0.05 versus value of WT (analysis of variance (ANOVA));#P<0.05 versus value of Atg5−/−(ANOVA); ‘NS’ indicates not significant versus value of WT (ANOVA). Figure 4: Clearance of mitochondria by macroautophagy from reticulocytes of WT and Atg5 −/− mice, but not Ulk1 gt/gt or DKO mice. ( a – f ) Representative EM of WT ( a ), ATG5 −/− ( b ), Ulk1 gt/gt ( c , d ) and DKO ( e , f ) reticulocytes from embryonic liver (E14.5). ( a , b ) Mitophagy was detected in WT and ATG5 −/− cells (scale bar, 1 μm). Insets indicate mitophagy (scale bar, 0.2 μm). ( c , e ) In Ulk1 gt/gt and DKO cells, numerous mitochondria were in contact with membrane structures (scale bar, 1 μm). Enlarged images are shown on the right side (scale bar, 0.2 μm). ( d , f ) Some Ulk1 gt/gt and DKO cells showed plasma membrane blebs containing mitochondria (scale bar, 1 μm). ( g , h ) Quantitative analysis of mitophagy calculated from EM photos in the embryonic liver at E18.5. Population of reticulocytes with mitophagy ( g ), and number of mitochondria per reticulocytes ( h ) were calculated ( n >35 cells per mouse). The data are shown as mean±s.d. ( n =3). * P <0.05 versus value of WT (analysis of variance (ANOVA)); # P <0.05 versus value of Atg5 −/− (ANOVA); ‘NS’ indicates not significant versus value of WT (ANOVA). Full size image To address the molecular mechanisms of mitophagy during erythrocyte differentiation, erythroblasts (EB; mitochondria high Syto16 high cells) and reticulocytes (RC; mitochondria high Syto16 low cells) were isolated from embryonic liver using Ter119-conjugated beads, followed by flow cytometric cell sorting. EC (Ter119-positive cells) were also purified from peripheral blood using Ter119-conjugated beads. The expression of key mitochondrial proteins was examined by western blotting. The mitochondrial outer membrane proteins, Tom20 and VDAC, were absent in EC from WT embryos due to mitochondrial clearance. They were detected at low levels in Atg5 −/− EC and at high levels in Ulk1 gt/gt and DKO EC ( Fig. 5a,b ). These data confirmed the partial impairment of mitochondrial clearance in Atg5 −/− and severe impairment in Ulk1 gt/gt and DKO EC. The protein Nix was recently identified as a selective autophagy receptor responsible for mitochondrial clearance from reticulocytes [19] , [20] , [21] , [22] . Accordingly, the expression level of Nix in these cell types was proportional to the extent of mitophagy ( Fig. 5a,b ; EC). Conventional macroautophagy was detected in WT and Ulk1 gt/gt , but not in Atg5 −/− and DKO, erythroblasts and reticulocytes, based on the levels of LC3-II and p62 ( Fig. 5a,b ). However, this process may not be involved in mitochondrial clearance because mitophagy occurred in Atg5 −/− cells where conventional macroautophagy was absent. Furthermore, most signals for LC3 (conventional macroautophagy marker) did not co-localize with Tom20 signals (mitochondria marker) in the erythroblasts and early reticulocytes of WT and Ulk1 gt/gt embryos ( Supplementary Fig. 6 ). Therefore, conventional macroautophagy would not contribute to mitochondrial clearance from fetal definitive reticulocytes. 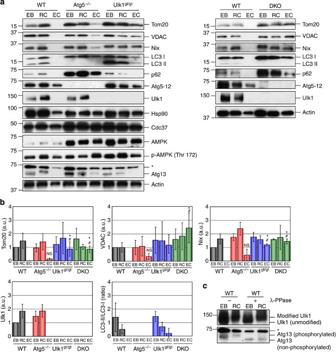Figure 5: Expression of autophagy-related proteins during erythrocyte differentiation. (a) Erythroblasts (EB; mitochondriahighSyto16high), reticulocytes (RC; mitochondriahighSyto16low) and EC (EC; Ter119+PBC) were collected from the indicated embryos (E18.5), and the expression of each protein was examined by western blot. The asterisk indicates a nonspecific band. Uncropped images are shown inSupplementary Figs 11 and 12. (b) Semi-quantitative analysis of the expression level of each protein and the LC3-II/LC3-I ratio (mean±s.d.,n=3). *P<0.05 versus value of WT EC (analysis of variance (ANOVA));#P<0.05 versus value of Atg5−/−EC (ANOVA); ‘NS’ indicates not significant versus value of WT EC (ANOVA). (c) Modification of Ulk1 and Atg13 during erythrocyte maturation. Cell lysates were treated withλ-phosphatase (400 U) for 45 min at 30 °C, and band shift was examined by anti-Ulk1 and anti-Atg13 antibodies. Asterisk indicates non-specific band. Uncropped images are shown inSupplementary Fig. 12. Figure 5: Expression of autophagy-related proteins during erythrocyte differentiation. ( a ) Erythroblasts (EB; mitochondria high Syto16 high ), reticulocytes (RC; mitochondria high Syto16 low ) and EC (EC; Ter119 + PBC) were collected from the indicated embryos (E18.5), and the expression of each protein was examined by western blot. The asterisk indicates a nonspecific band. Uncropped images are shown in Supplementary Figs 11 and 12 . ( b ) Semi-quantitative analysis of the expression level of each protein and the LC3-II/LC3-I ratio (mean±s.d., n =3). * P <0.05 versus value of WT EC (analysis of variance (ANOVA)); # P <0.05 versus value of Atg5 −/− EC (ANOVA); ‘NS’ indicates not significant versus value of WT EC (ANOVA). ( c ) Modification of Ulk1 and Atg13 during erythrocyte maturation. Cell lysates were treated with λ -phosphatase (400 U) for 45 min at 30 °C, and band shift was examined by anti-Ulk1 and anti-Atg13 antibodies. Asterisk indicates non-specific band. Uncropped images are shown in Supplementary Fig. 12 . Full size image The WT and Atg5 −/− reticulocytes expressed a high molecular weight Ulk1 isoform, compared with their erythroblasts ( Fig. 5a ). Ulk1 is regulated by posttranslational modifications such as phosphorylation [8] , [9] and acetylation [10] . Since the Ulk1 modification in reticulocytes was not changed by phosphatase treatment ( Fig. 5c ), Ulk1 acetylation, but not phosphorylation, seems to be crucial for mitochondrial clearance, although the possibility was not excluded that unidentified modification occurs in Ulk1. Although Hsp90, Cdc37 and AMPK were recently found responsible for Ulk1 activation [8] , [9] , these proteins were slightly upregulated in WT reticulocytes, but not in Atg5 −/− reticulocytes ( Fig. 5a ) despite the occurrence of mitophagy. In addition, a downstream effector of Ulk1 (Atg13) may be phosphorylated in WT reticulocytes (based on phosphatase reaction ( Fig. 5c )), but not in Atg5 −/− reticulocytes ( Fig. 5a ). These data support the existence of an unidentified Ulk1-mediated signalling pathway promoting cell differentiation in Atg5 −/− reticulocytes. Mitochondrial removal by alternative macroautophagy in vitro The involvement of alternative macroautophagy in mitochondrial clearance during erythrocyte maturation was further confirmed using an in vitro erythrocyte differentiation system. Nascent erythroblasts were purified from the liver of E14.5 embryos and cultured in erythrocyte differentiation medium (see Methods). Three days after the induction of differentiation, >60% of the cells had lost their nuclei and become reticulocytes in every genotype ( Fig. 6a,b ). Thereafter, the enucleated cells (Syto16 low cells) lost their mitochondria in the cultures of WT cells, as shown by a gradual increase in the number of mitochondria low Syto16 low cells (mature red blood cells) ( Fig. 6c,d ). Similar results were obtained with Atg5 −/− erythroid cells. In contrast, the number of mitochondria low Syto16 low cells did not increase in Ulk1 gt/gt and DKO cells ( Fig. 6c,d ), indicating that Ulk1 is essential for mitochondrial clearance during in vitro differentiation, which is consistent with the in vivo findings. Wortmannin and 3-methyladenine are frequently used autophagy inhibitors known to inhibit both conventional and alternative macroautophagy [6] . The addition of these inhibitors to the cultures of WT cells almost completely suppressed mitochondrial clearance from Syto16 low cells ( Fig. 6e,f ). These autophagy inhibitors also suppressed mitochondrial clearance in Atg5 −/− cells ( Fig. 6i ), indicating this process was dependent on alternative macroautophagy. In contrast, rapamycin (conventional macroautophagy inducer) and compound C (AMPK inhibitor) did not have any effect ( Fig. 6g,h ). These data collectively indicate that alternative macroautophagy is responsible for mitochondrial clearance from embryonic reticulocytes. 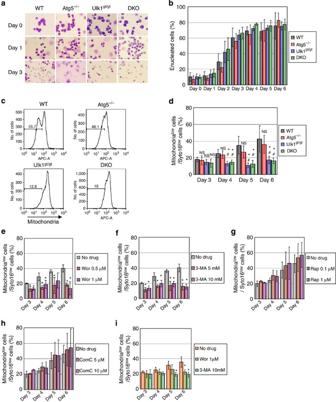Figure 6: Role of alternative macroautophagy in mitochondrial clearance during erythrocyte differentiationin vitro. (a) Morphology of cultured erythroid cells on day 0, 1 and 3 of differentiation. Erythroblasts were purified from embryonic liver (E14.5) and incubated for the indicated times in erythrocyte differentiation medium. The cells were stained with a Diff-quick kit. (b) Percentage of cells without nuclei (Syto16lowcells) on the indicated days of differentiation (mean±s.d.,n=6). Loss of nuclei occurred normally in all mice. (c,d) Percentage of Syto16lowcells without mitochondria. Differentiated cells were stained with Syto16 and Mitotracker Deep Red. Representative histograms of mitochondrial content in Syto16lowcells on day 6 are shown in (c). Numbers indicate the population of mitochondrialowcells. Representative dot plots are also available inSupplementary Fig. 13. (d) Percentage of Syto16lowcells lacking mitochondria determined by gating the mitochondrialowfraction as shown in (c) (mean±s.d.,n=6). *P<0.05 versus value of WT (analysis of variance (ANOVA));#P<0.05 versus value of Atg5−/−(ANOVA); ‘NS’ indicates not significant versus value of WT (ANOVA). (e–h) Impact of various drugs on mitochondrial clearance duringin vitrodifferentiation. Differentiated cells from WT embryos were incubated with or without wortmannin (e), 3-methyladenine (3-MA) (f), rapamycin (g) or compound C (h) at the indicated concentrations and time periods. Percentage of mitochondrialowcells/Syto16lowcells was measured by flow cytometry (mean±s.d.,n=3). *P<0.05 versus value of no drug (ANOVA). (i) Similar experiments were performed with cells from Atg5−/−embryos exposed to wortmannin or 3-MA (mean±s.d.,n=3). *P<0.05 versus value of no drug (ANOVA). Figure 6: Role of alternative macroautophagy in mitochondrial clearance during erythrocyte differentiation in vitro . ( a ) Morphology of cultured erythroid cells on day 0, 1 and 3 of differentiation. Erythroblasts were purified from embryonic liver (E14.5) and incubated for the indicated times in erythrocyte differentiation medium. The cells were stained with a Diff-quick kit. ( b ) Percentage of cells without nuclei (Syto16 low cells) on the indicated days of differentiation (mean±s.d., n =6). Loss of nuclei occurred normally in all mice. ( c , d ) Percentage of Syto16 low cells without mitochondria. Differentiated cells were stained with Syto16 and Mitotracker Deep Red. Representative histograms of mitochondrial content in Syto16 low cells on day 6 are shown in ( c ). Numbers indicate the population of mitochondria low cells. Representative dot plots are also available in Supplementary Fig. 13 . ( d ) Percentage of Syto16 low cells lacking mitochondria determined by gating the mitochondria low fraction as shown in ( c ) (mean±s.d., n =6). * P <0.05 versus value of WT (analysis of variance (ANOVA)); # P <0.05 versus value of Atg5 −/− (ANOVA); ‘NS’ indicates not significant versus value of WT (ANOVA). ( e – h ) Impact of various drugs on mitochondrial clearance during in vitro differentiation. Differentiated cells from WT embryos were incubated with or without wortmannin ( e ), 3-methyladenine (3-MA) ( f ), rapamycin ( g ) or compound C ( h ) at the indicated concentrations and time periods. Percentage of mitochondria low cells/Syto16 low cells was measured by flow cytometry (mean±s.d., n =3). * P <0.05 versus value of no drug (ANOVA). ( i ) Similar experiments were performed with cells from Atg5 −/− embryos exposed to wortmannin or 3-MA (mean±s.d., n =3). * P <0.05 versus value of no drug (ANOVA). Full size image Mitophagy in primitive and adult definitive reticulocytes The contribution of Ulk1-dependent alternative macroautophagy was assessed in the other two waves of erythroid lineage: the primitive- and adult definitive lineages. The primitive wave emerges within the yolk sac blood islands [23] . The role of Ulk1 in mitochondrial clearance was examined in primitive erythrocyte by analysing whole blood in embryo at E11.5. Enucleation and mitochondrial clearance in Ulk1 gt/gt erythroid cells were normally induced, as assessed by Syto16 and Mitotracker Deep Red staining, respectively ( Supplementary Fig. 7 ). Therefore Ulk1 is not involved in the maturation of first primitive erythroid cells. Adult definitive erythroid cells were investigated using Atg7 F/F Cre adult mice exhibiting abnormal mitochondrial clearance during erythrocyte maturation [18] . We hypothesized that adult and embryonic Atg7 F/F Cre mice express distinct mechanisms of mitochondrial clearance. To test this possibility, we compared peripheral blood cells (PBC) from WT, Ulk1 gt/gt and Atg7 F/F Cre adult mice. The Atg7 F/F Cre mice exhibited the typical severe anaemia ( Fig. 7a ) as previously reported. This is likely due to a failure of early stage erythrocyte differentiation because the bone marrow Sca1 − c-Kit + progenitors were severely downregulated ( Fig. 7b ), as previously reported [22] . Analysis of circulating EC indicated that the population of mitochondria-containing Ter119 + cells was higher in Atg7 F/F Cre mice and Ulk1 gt/gt mice than in WT mice ( Fig. 7c ), but the population of mitochondria high Ter119 + cells accounted for only 10% of all cells in both mice, which was considerably lower than those in the embryos. Similar results were obtained when the mitochondria-containing cells were counted among the Syto16 low cells ( Fig. 7d ). Furthermore, mitophagy was detected in bone marrow erythroid cells of Ulk1 gt/gt mice ( Fig. 7e ). Based on western blot analysis, mitochondrial clearance was almost normal in the bone marrow erythroid cells of Ulk1 gt/gt mice ( Fig. 7f,g ). These data indicate that the effect of Ulk1 and Atg7 on mitochondrial clearance from adult definitive reticulocytes was far less prominent than in fetal definitive reticulocytes. 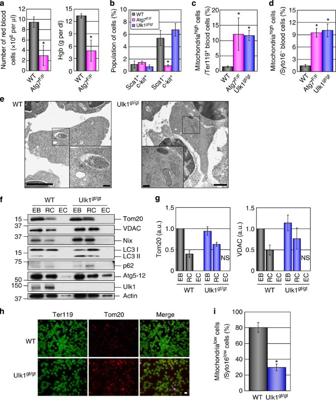Figure 7: Analysis of mitochondrial clearance during adult erythropoiesis. (a) Number of EC and haemoglobin content in the blood of the indicated mice (10–20 weeks old; mean±s.d.,n=6). *P<0.05 versus value of WT (Student'st-test). (b) Analysis of early erythrocyte development. Bone marrow cells were harvested from the indicated mice (10–20 weeks old) and stained with anti-cKit and anti-Sca1 antibodies. The population of each cell type was counted by FACS (mean±s.d.,n=3). *P<0.05 versus value of WT (analysis of variance (ANOVA)). (c) Percentage of mitochondria-containing Ter119+blood cells. Cells in peripheral blood from the indicated mice (10–20 weeks old) were stained with anti-Ter119 antibody together with Mitotracker Deep Red. The population of mitochondriahighcells among Ter119-positive cells was counted by FACS (mean±s.d.,n=3). *P<0.05 versus value of WT (ANOVA). (d) Percentage of mitochondria-containing Syto16lowblood cells. Cells in peripheral blood from the indicated mice (10–20 weeks old) were stained with Syto16 and Mitotracker Deep Red. The population of mitochondriahighcells among Syto16-negative cells was counted by FACS (mean±s.d.,n=3). *P<0.05 versus value of WT (ANOVA). (e) Representative electron micrographs of bone marrow reticulocytes in 10 week-old WT and Ulk1gt/gtmice (scale bar, 1 μm). Insets indicate mitophagy (scale bar, 0.2 μm). (f,g) Erythroblasts (EB; mitochondriahighSyto16high), reticulocytes (RC; mitochondriahighSyto16low) and EC (EC; Ter119+PBC) were collected from the indicated mice (10–20 weeks old), and the expression of each protein was examined by western blot. Uncropped images are shown inSupplementary Fig. 14. (g) Semi-quantitative analysis of the expression level of each protein (mean±s.d.,n=3). ‘NS’ indicates not significant versus value of WT EC (ANOVA). (h,i) The impact of Ulk1 on mitochondrial clearance during stress erythropoiesis. (h) Representative images of erythrocyte in PHZ-treated WT and Ulk1gt/gtmice (14 weeks old). Blood cells were stained with anti-Ter119 (erythroid cell marker) and anti-Tom20 (mitochondrial marker) antibodies and observed by fluorescence microscopy. Green and red indicate Ter119 and Tom20, respectively. Scale bar, 10 μm. (i) Percentage of mitochondrialowcells among Syto16lowcells. Erythroid cells were stained with Syto16 (DNA) and Mitotracker Deep Red (mean±s.d.,n=3). *P<0.05 versus value of WT (Student’st-test). Mitochondrial retention was observed in Ulk1gt/gtmice. Figure 7: Analysis of mitochondrial clearance during adult erythropoiesis. ( a ) Number of EC and haemoglobin content in the blood of the indicated mice (10–20 weeks old; mean±s.d., n =6). * P <0.05 versus value of WT (Student's t -test). ( b ) Analysis of early erythrocyte development. Bone marrow cells were harvested from the indicated mice (10–20 weeks old) and stained with anti-cKit and anti-Sca1 antibodies. The population of each cell type was counted by FACS (mean±s.d., n =3). * P <0.05 versus value of WT (analysis of variance (ANOVA)). ( c ) Percentage of mitochondria-containing Ter119 + blood cells. Cells in peripheral blood from the indicated mice (10–20 weeks old) were stained with anti-Ter119 antibody together with Mitotracker Deep Red. The population of mitochondria high cells among Ter119-positive cells was counted by FACS (mean±s.d., n =3). * P <0.05 versus value of WT (ANOVA). ( d ) Percentage of mitochondria-containing Syto16 low blood cells. Cells in peripheral blood from the indicated mice (10–20 weeks old) were stained with Syto16 and Mitotracker Deep Red. The population of mitochondria high cells among Syto16-negative cells was counted by FACS (mean±s.d., n =3). * P <0.05 versus value of WT (ANOVA). ( e ) Representative electron micrographs of bone marrow reticulocytes in 10 week-old WT and Ulk1 gt/gt mice (scale bar, 1 μm). Insets indicate mitophagy (scale bar, 0.2 μm). ( f , g ) Erythroblasts (EB; mitochondria high Syto16 high ), reticulocytes (RC; mitochondria high Syto16 low ) and EC (EC; Ter119 + PBC) were collected from the indicated mice (10–20 weeks old), and the expression of each protein was examined by western blot. Uncropped images are shown in Supplementary Fig. 14 . ( g ) Semi-quantitative analysis of the expression level of each protein (mean±s.d., n =3). ‘NS’ indicates not significant versus value of WT EC (ANOVA). ( h , i ) The impact of Ulk1 on mitochondrial clearance during stress erythropoiesis. ( h ) Representative images of erythrocyte in PHZ-treated WT and Ulk1 gt/gt mice (14 weeks old). Blood cells were stained with anti-Ter119 (erythroid cell marker) and anti-Tom20 (mitochondrial marker) antibodies and observed by fluorescence microscopy. Green and red indicate Ter119 and Tom20, respectively. Scale bar, 10 μm. ( i ) Percentage of mitochondria low cells among Syto16 low cells. Erythroid cells were stained with Syto16 (DNA) and Mitotracker Deep Red (mean±s.d., n =3). * P <0.05 versus value of WT (Student’s t -test). Mitochondrial retention was observed in Ulk1 gt/gt mice. Full size image Finally, we tested the contribution of Ulk1 to mitochondrial clearance during stress erythropoiesis. Acute anaemic stress triggers the rapid accumulation of new EC by a process distinct from steady-state erythropoiesis, and resembling the one of fetal definitive erythroid cells. Stress erythropoiesis was induced in vivo by injecting WT and Ulk1 gt/gt mice with the haemolytic agent phenylhydrazine (PHZ) [24] . These mice showed significant and comparable reductions in the number of circulating EC, compared with untreated mice ( Supplementary Fig. 8 ). Mitochondrial clearance was less efficient in PHZ-treated Ulk1 gt/gt mice than in PHZ-treated WT mice ( Fig. 7h,i ), unlike steady-state erythropoiesis. These data suggest that Ulk1-dependent alternative macroautophagy is also involved in stress erythropoiesis. The present study demonstrated the contributions of alternative macroautophagy to mitochondrial clearance during the differentiation of EC. The main findings are as follows: First, mitochondrial clearance from reticulocytes occurs mainly by Ulk1-dependent Atg5-independent alternative macroautophagy in fetal definitive erythroid cells. Second, the impact of Ulk1 on mitochondrial clearance is markedly reduced in adult mice. Third, Atg7 F/F Cre mice exhibited severe anaemia; this anaemia was probably due to abnormal early differentiation as reported previously [25] . These findings support a new physiological role for Ulk1-dependent alternative macroautophagy during erythrocyte development, and the existence of Ulk1-independent processes in mature mammals. The role of Ulk1 in mitochondrial clearance from reticulocytes was previously described [8] , [11] , but the molecular mechanisms have not been elucidated. Because Ulk1 was described as an initiator of conventional Atg5/Atg7-dependent macroautophagy, it is generally believed that mitochondria are digested by conventional macroautophagy. However, we recently discovered that mammalian cells conduct Atg5-independent macroautophagy largely regulated by Ulk1 (ref. 6 ). Therefore, we hypothesized that Ulk1-dependent Atg5-independent macroautophagy plays a role in mitochondrial clearance during erythrocyte differentiation, and found that mitophagy was detected in WT and Atg5 −/− reticulocytes, but not in Ulk1 gt/gt and DKO reticulocytes. We also demonstrated that mitochondria were retained in mature erythroid cells of Ulk1 gt/gt and DKO embryos and the inhibition of alternative macroautophagy almost completely prevented mitochondrial clearance from Atg5 −/− EC in vitro . In accordance, we concluded that the lack of Atg5 had less effect on mitophagy than the lack of Ulk1. These results indicate that Ulk1 is crucial for mitochondrial clearance via alternative macroautophagy. What are the signalling pathways implicated in alternative Ulk1-mediated Atg5-independent macroautophagy? The contribution of conventional Ulk1 effectors (that is, Hsp90, Cdc37, AMPK and Atg13) is unlikely because we have shown that modifications of these proteins were not correlated with mitophagy in Atg5 −/− reticulocytes ( Fig. 5 ). In contrast, Nix expression levels correlated with mitophagy in all mouse genotypes. Nix was reported to have a function for the partial elimination of mitochondria via conventional macroautophagy [19] , [20] , [21] , and also found crucial for LC3-independent mitophagy [22] . The latter machinery may be identical to alternative macroautophagy. Therefore, Nix seems to be involved in the mitophagy mediated by both conventional and alternative macroautophagy. Note that our current data only proposes the possible involvement of Nix, and future studies will be required to identify the molecular mechanisms of mitophagy including Nix dependency. Mice with organ-specific Atg5 and Atg7 deficiency show various abnormalities, indicating that conventional macroautophagy is crucial for organ development and homeostasis [26] , [27] . Therefore, why does alternative macroautophagy, and not conventional macroautophagy, have an essential role in fetal definitive erythrocyte maturation? One possible explanation would be that alternative macroautophagy is only activated in Atg5-deficient cells as a compensation mechanism for conventional macroautophagy. However, this explanation is not supported by the poor colocalization of LC3 and Tom20 in WT reticulocytes ( Supplementary Figs 3 and 6 ). Another possibility would be the lack of proteins or lipids required for conventional macroautophagy in embryonic reticulocytes. However, this is also unlikely because conventional macroautophagy was observed in WT and Ulk1 gt/gt reticulocytes ( Fig. 5 ; immunoblot of p62 and LC3). A more plausible explanation would be that conventional and alternative macroautophagy are supported by distinct machineries activated by different stimuli, and the alternative macroautophagy is the dominant force of mitochondrial clearance during fetal definitive erythropoiesis. Further studies will be required to identify the stimuli and conditions specific for conventional and alternative macroautophagy. The present study also showed the data about mitochondrial clearance from adult definitive erythroid cells. Although engulfment and digestion of mitochondria by autophagic vacuoles were clearly observed in EC of adult mice ( Fig. 7e ), Atg7 and Ulk1 did not have an important role in this process. The involvement of the Ulk1 homologue, Ulk2, was ruled out because it is not expressed by erythroid cells in adult mice ( Supplementary Fig. 9 ). Therefore, Ulk1/Ulk2-independent Atg5/Atg7-independent macroautophagy may occur in adult EC. In conclusion, this study demonstrates that mitochondrial clearance by Ulk1-dependent Atg5-independent alternative macroautophagy is essential for erythrocyte differentiation during fetal definitive erythrocytosis, but not in mature mammals. The specific activation during organ development suggests that this process is supported by signalling machinery distinct from that of conventional Atg5/Atg7-dependent macroautophagy. Elucidation of these signalling pathways may lead to the identification of genetic markers of congenital haematologic diseases. Generation of Ulk1 gt/gt mice To generate Ulk1 gene trap mice, the ES cell line targeting the ulk1 gene was purchased from the Texas A&M Institute for Genomic Medicine (TIGM; College Station, TX, USA). The gene trap vector 48 (VICTR48) was inserted into intron 3 ( Supplementary Fig. 1 ). The ES cell clones were microinjected into blastocysts to generate gene trap chimeras. The chimeric mice were screened for the presence of the β-geo gene trap cassette. Gene trap-positive chimeras were intercrossed with C57BL/6 mice for at least eight generations. The Atg5 −/− and Atg7-flox mice were described in other studies [28] , [29] . The vav1-cre mice were purchased from the Jackson Laboratory (Bar Harbor, ME, USA). All animal experiments were approved by the Institutional Animal Care and Use Committee of the Tokyo Medical and Dental University. Mice were bred at the Laboratory for Recombinant Animals (Medical Research Institute, Tokyo Medical and Dental University, Tokyo, Japan). Antibodies and chemicals The following polyclonal antibodies were used for immunoblot and immunofluorescence assays: anti-Ulk1 (Sigma-Aldrich, #A7481; 1:1,000), anti-Atg5 (Sigma-Aldrich, #A0731; 1:1,000), anti-p62 (MBL, #PM045; 1:1,000), anti-Tom20 (Santa Cruz, #sc-11415; WB: 1:2,500, IF: 1:500), anti-Hsp90 (CST, #4877; 1:1,000), anti-VDAC (CST, #4866; 1:1,000), anti-AMPK (CST, #2532; 1:1,000) and anti-phospho-AMPK (CST, #2971; 1:1,000). The following monoclonal antibodies were also used: anti-Atg13 (MBL, #M183-3; 1:1,000), anti-Cdc37 (Santa Cruz, #sc-13129; 1:300), anti-LAMP2 (Abcam, #ab13524; 1:100), anti-Ter119 (BD Biosciences, #553670; 1:200), anti-NIX (CST, #12396; 1:1,000)), anti-LC3 (NanoTools, #0231; WB 1:1,000), anti-LC3 (Cosmobio, #CTB-LC3-2-1C; IF: 1:100), and anti-Actin (Millipore, #MAB1501; 1:2,500). Flow cytometry was conducted with fluorescein isothiocyanate (FITC)-labelled anti-CD71 (BD Biosciences, #553266; 1:200), PE-labelled anti-Ter119 (BD Biosciences, #553673; 1:200), FITC-labelled anti-Sca1 (BD Biosciences, #557405; 1:200) and PE-labelled anti-cKit (BD Biosciences, #553355; 1:200) antibodies. The chemicals 3-methyladenine, rapamycin and compound C were obtained from Sigma-Aldrich, Santa Cruz and Calbiochem, respectively. Mitotracker Deep Red (#M22426), Syto-16 (#S7578) and DAPI (#P36935) were purchased from Molecular Probes. SCF (#250-03) and insulin-like growth factor-1 (#100-11) were obtained from PeproTech, whereas dexamethasone (#D2915), holo-Transferrin (#T1283) and PHZ (#P26252) were obtained from Sigma-Aldrich. Recombinant human erythropoietin (EPO; #HZ-1021) and recombinant human insulin (#O105) were obtained from HumanZyme and CSTI, respectively. The other chemicals were purchased from Nacalai Tesque (Tokyo, Japan). Cell isolation Ter119-positive erythroid lineage cells were isolated from mouse liver at embryonic day 18.5 (E18.5) using magnetic beads conjugated with anti-Ter119 antibody (BD IMag cell separation system). Erythroblasts (mitochondria high Syto16 high ) and reticulocytes (mitochondria high Syto16 low ) were isolated by cell sorting using a FACS Aria II (BD Biosciences). EC were collected from the peripheral blood using the IMag cell separation system. Immunoblot analysis Cell samples were homogenized in SDS sample buffer and loaded on SDS-polyacrylamide gels. The protein bands were transferred to polyvinylidene difluoride membranes (Millipore). The membranes were blocked with 3% skim milk in TBS containing 0.1% Tween-20 (TBS-T), and then incubated with the primary antibody overnight at 4 °C. After washes in TBS-T, the membranes were incubated with the horseradish peroxidase-labelled secondary antibody and visualized with Chemi-Lumi One Super reagent. Protein band density was semi-quantified using ImageJ software. Protein dephosphorylation of Ulk1 and Atg13 was conducted by incubating cell lysates with 400 U λ-phosphatase (45 min; 30 °C) and band shift was examined by western blot analysis. All experiments were conducted at least in triplicates. We supplied several uncropped scans of the western blots in Supplementary Figures . Immunofluorescence analysis Cells were fixed in 4% paraformaldehyde, pelleted on slides by cytospin3 (Shandon), and stained with primary antibodies for 1 h at room temperature. After washes, the cells were stained with secondary antibodies, mounted in ProLong Gold antifade reagent with DAPI, and examined by confocal microscopy (LSM510 Zeiss). Electron microscopy Cells were fixed with 1.5% paraformaldehyde/3% glutaraldehyde in 0.1 M phosphate buffer (pH 7.3), followed by 1% OsO 4 . After dehydration, the fixed cells were embedded in Epon812. Thin sections were cut and stained with uranyl acetate lead citrate for observation under a JEM-1010 electron microscope (JEOL Co. Ltd.) at 80 k. Analysis of erythroid differentiation Erythroid cells were obtained from the liver and peripheral blood of embryonic E18.5 mice. Hepatic erythroid cells were isolated from liver tissue using a 70-μm cell strainer. Erythroid cells were also obtained from the bone marrow and peripheral blood of adult mice. For three-colour analysis of erythrocyte differentiation and mitochondria, the cells were incubated with PE-conjugated anti-Ter119, FITC-conjugated anti-CD71 antibody, and Mitotracker Deep Red (30 min; 4 °C). For two-colour analysis of nuclei and mitochondria, the cells were incubated with Syto-16 and Mitotracker Deep Red (30 min; 4 °C). For the analysis of early erythrocyte differentiation, bone marrow cells were incubated with PE-conjugated anti-cKit and FITC-conjugated anti-Sca1 antibody (30 min; 4 °C). Stained cells were washed with PBS and analysed by flow cytometry with a FACS CantII (BD Biosciences). Data analysis was performed with BD FACSDiva and Flowjo software. In vitro erythroid differentiation Erythroblasts were purified from embryonic mouse liver (E14.5), and then suspended at 1 × 10 6 cells ml −1 in a 24-well gelatin-coated tissue culture dish containing StemPro34 plus Nutrient Supplement (Invitrogen) with 2 units ml −1 of human EPO, 100 ng ml −1 of SCF, 10 −6 M dexamethasone, 40 ng ml −1 of insulin-like growth factor-1 and penicillin/streptomycin. After 1 or 3 days of culture, the nonadherent cells were collected, filtered through a 70-μm cell strainer and transferred to a fresh gelatin-coated dish for the induction of differentiation as follows. In brief, erythroblasts were washed with PB2 buffer (0.1% glucose and 0.3% bovine serum albumin in PBS), and suspended in Iscove’s modified Dulbecco’s medium containing 15% fetal bovine serum, 1% detoxified bovine serum albumin, 200 μg ml −1 of holo-Transferrin, 10 μg ml −1 of recombinant human insulin, 2 mM L -glutamine, 10 −4 M β-mercaptoethanol and 2 units ml −1 of EPO. The cultures were examined after staining with a Diff-quick staining kit (Sysmex). Various agents were added on day 2 to assess their effects on cell differentiation. Mitochondrial clearance was examined by flow cytometry after staining with Syto-16 and Mitotracker Deep Red. Stress hematopoiesis Mice were injected subcutaneously with PHZ [24] (50 mg kg −1 in sterile saline). After 7 days, they were killed and blood was collected from the caudal vena cava. Isolation of primitive erythrocyte After removal of the placenta, embryos were transferred to dishes containing heparinized PBS. Blood cells were collected by aspiration as they bled. Haematology tests Peripheral blood samples were harvested in heparinized tubes, and analysed with a blood cell counter (ERMA Inc.) using the programme for mice. Statistical analysis Results are expressed as the mean±s.d. Statistical evaluation was performed using Prism (GraphPad) software. Comparisons of two data sets were performed using unpaired two-tailed Student’s t -test. All other comparisons of multiple data sets were performed using one-way analysis of variance followed by Tukey's post hoc test. Statistical significance was established for P -values of <0.05. How to cite this article : Honda, S. et al . Ulk1-mediated Atg5-independent macroautophagy mediates elimination of mitochondria from embryonic reticulocytes. Nat. Commun. 5:4004 doi: 10.1038/ncomms5004 (2014).